Small RNA mediated gradual control of lipopolysaccharide biosynthesis affects antibiotic resistance inHelicobacter pylori The small, regulatory RNA RepG ( Re gulator of p olymeric G -repeats) regulates the expression of the chemotaxis receptor TlpB in Helicobacter pylori by targeting a variable G-repeat in the tlpB mRNA leader. Here, we show that RepG additionally controls lipopolysaccharide (LPS) phase variation by also modulating the expression of a gene ( hp0102 ) that is co-transcribed with tlpB . The hp0102 gene encodes a glycosyltransferase required for LPS O-chain biosynthesis and in vivo colonization of the mouse stomach. The G-repeat length defines a gradual (rather than ON/OFF) control of LPS biosynthesis by RepG, and leads to gradual resistance to a membrane-targeting antibiotic. Thus, RepG-mediated modulation of LPS structure might impact host immune recognition and antibiotic sensitivity, thereby helping H. pylori to adapt and persist in the host. Lipopolysaccharide (LPS) is essential for the physiological integrity and functionality of the outer membrane of most Gram-negative bacteria. As a main surface antigen, it also plays an important role in the interaction between bacterial pathogens and their host. LPS is one of the most potent stimulators of the host immune system and its recognition is essential for the host organism to clear bacterial infections [1] . During the course of infection, many pathogens modify their LPS synthesis and structure to adapt to diverse microenvironments and evade recognition by the host’s immune system [2] . Helicobacter pylori is a Gram-negative pathogen that colonizes the stomach of 50% of the world’s population, which can lead to peptic ulcer disease and gastric cancer [3] . H. pylori produces a highly modified LPS, unique in both its structure and function, that is essential for establishing colonization and persistence within the human stomach [4] , [5] , [6] . Like in most Gram-negative bacteria, H. pylori LPS is composed of lipid A, a core oligosaccharide, and the hypervariable O-specific polysaccharide repeats (O-chain) [7] . H. pylori LPS lacks a canonical inner and outer core organization, and was recently reported to have a short core and a longer O-antigen domain, including structures that were previously assigned to the outer core [8] . This long O-antigen comprises a trisaccharide (Trio), a glucan, a DD-heptan, and terminal Lewis antigens. Despite its important roles in immune evasion and persistence, a complete picture of the LPS biosynthesis pathway in H. pylori is only being revealed stepwise [4] , [9] , [10] . This might be due to the dispersed genomic locations of LPS genes throughout the H. pylori genome. Compared to enterobacterial LPS, H. pylori LPS has a reduced immunostimulatory effect (~1,000-fold reduced) due to an under-acetylated and dephosphorylated lipid A [2] . Moreover, the H. pylori O-chain contains fucosylated oligosaccharides that mimic the structure of mammalian histo-blood group antigens, including Lewis x/y antigens [2] , [5] . Both the low endotoxicity of the lipid A and the molecular mimicry of human Lewis antigens contribute to H. pylori host immune surveillance and establishment of long-lasting infection [7] , [11] , [12] . H. pylori LPS is highly variable [13] . Phase-variable ON/OFF expression of LPS biosynthetic genes, such as Lewis antigen-producing fucosyltransferases, has been shown to increase the diversity of LPS phenotypes, thereby enabling H. pylori to adapt to its individual host and/or changing environments in the gastric mucosa during infection [14] , [15] . Different H. pylori clinical isolates were found to extensively alter their Lewis antigen expression in vivo, probably reflecting bacterial adaptation to intra-individual host environments [16] . Hypervariable simple sequence repeats (SSRs) are a major source of so-called phase variation, which facilitates adaptation to changing environments and immune escape of pathogens [17] , [18] . Length variation of SSRs occurring during replication can either affect translation through the introduction of frameshift mutations (intragenic) or transcription (intergenic) by changing the spacing of promoter elements or transcription factor binding sites [17] . We previously uncovered that SSRs can also serve as targeting sites for small regulatory RNAs (sRNAs), an important class of post-transcriptional regulators controlling gene expression in response to various stress conditions or during infection [19] , [20] . We previously demonstrated that the conserved and abundant H. pylori sRNA RepG ( Re gulator of p olymeric G -repeats) directly base-pairs with its C/U-rich terminator loop to a phase-variable homopolymeric G-repeat in the 5′ untranslated region (UTR) of the tlpB mRNA, encoding the chemotaxis receptor TlpB [21] . The length of this SSR determines the outcome of post-transcriptional control (activation/repression) of TlpB by RepG and thereby gradually modulates tlpB expression. Although TlpB is assumed to play a role in quorum sensing, biofilm dispersal, acid-/urea-sensing, and pH-taxis [22] , [23] , [24] , [25] , its role in host colonization by H. pylori is controversial [23] , [26] , [27] . Thus, the biological rationale of controlling TlpB via a variable SSR remained unclear. Using sequence conservation analysis, we noticed that H. pylori tlpB is typically encoded upstream of hp0102 , a gene with previously unknown function. Here, we show that the encoded HP0102 protein is required for LPS O-chain production as well as Lewis x antigen display and is essential for murine stomach colonization. Furthermore, we show that Δ hp0102 mutants display an increased sensitivity to high-salt stress and antibiotics treatment. Our study demonstrates that RepG co-regulates expression of tlpB and hp0102 , which are transcribed in a bicistronic mRNA, and that the length of the homopolymeric G-repeat in the tlpB-hp0102 leader determines the outcome of RepG-mediated control of tlpB-hp0102 mRNA. The post-transcriptional regulation of hp0102 expression by antisense base-pairing of a sRNA to a variable SSR allows for a gradual modulation of LPS biosynthesis as well as Lewis x antigen display, a more scalable mechanism than the previously reported ON/OFF control. In turn, the fine-tuning of LPS O-chain expression also mediates gradual resistance of H. pylori to a membrane-targeting antibiotic. Expression of the tlpB - hp0102 operon is regulated by RepG The H. pylori RepG sRNA directly interacts with a 12G-repeat in the 5′ UTR of tlpB mRNA and thereby post-transcriptionally represses tlpB in strain 26695 (Fig. 1a , ref. [21] ). RepG is highly conserved among different H. pylori strains, and homologs are also present in the related gastric Helicobacter species, H. acinonychis , H. cetorum , and H. mustelae [21] . Our previous dRNA-seq study [28] suggested tlpB is transcribed as a bicistronic mRNA together with its downstream gene hp0102 , which we could validate by RT-PCR analysis (Supplementary Fig. 1a, b ). We found a highly conserved genetic organization with adjacent tlpB and hp0102 genes in 86 H. pylori genomes (Supplementary Fig. 1c ). Notably, in the closely related H. acinonychis and H. cetorum species, the tlpB and hp0102 homologous genes are also adjacent and preceded by a G-repeat sequence. The conserved genetic organization of tlpB and hp0102 was suggestive of their co-expression and co-regulation by RepG. Fig. 1: RepG sRNA represses expression of the tlpB - hp0102 mRNA. a In H. pylori strain 26695, RepG sRNA is transcribed from the intergenic region between hp1043 and hp1044 , encoding an orphan response regulator and a protein of unknown function. The C/U-rich terminator loop of RepG (blue) binds to a homopolymeric G-repeat (12G, light gray) in the 5′ UTR of the bicistronic tlpB - hp0102 mRNA (dotted line), encoding a chemotaxis receptor and a protein of unknown function [21] . Transcriptional start sites (TSS, +1; ref. [28] ) and ribosome binding sites (RBS) are indicated by arrows and black bars, respectively. Numbers designate the distance to the tlpB start codon. A G-rich sequence (G hp0102 , orange) was identified in the tlpB - hp0102 IGR. b RT-qPCR analysis of RepG-dependent regulation of tlpB and hp0102 in H. pylori strain 26695 wildtype (WT), repG deletion (∆ repG ), and complementation (C RepG ) mutants. Wild-type mRNA levels of each gene were set to 1, and relative mRNA levels in mutants are shown as bars. Values are shown as mean ± standard deviations (s.d.) for n = 6 ( tlpB ; exception C RepG n = 3) and n = 4 ( hp0102 ) biologically independent experiments. ****—highly significant, p -value < 0.0001; ***—highly significant, p -value < 0.001; n.s.—not significant; Student’s t -test, two-tailed. Source data underlying ( b ) is provided as a Source data file. Full size image RT-qPCR analysis showed about eight- and ten-fold increase in mRNA levels of the tlpB and hp0102 genes, respectively, in the Δ repG mutant when compared to the wildtype (WT) of H. pylori strain 26695 (Fig. 1b ). This co-regulation is in line with tlpB and hp0102 being encoded in an operon. Complementation of the Δ repG mutant with ectopically expressed RepG under control of its native promoter from the neutral rdxA locus (C RepG ) restored wild-type mRNA levels of both genes. This indicates that not only tlpB , but also hp0102 is repressed by RepG in H. pylori strain 26695. RepG represses HP0102 by targeting an upstream G-repeat To investigate whether RepG also controls HP0102 protein synthesis, we used a translational gfpmut3 reporter system established in strain G27 [21] . Here, the first ten amino acids of the 26695 hp0102 coding region were fused to gfpmut3 and introduced together with tlpB , including native promoter (P tlpB ) and 5′ UTR (12G), into the rdxA locus of G27 ( tlpB - hp0102 , Fig. 2a ). HP0102::GFP protein levels were increased about two-fold upon repG deletion, demonstrating that RepG represses expression of HP0102 (Fig. 2b and Supplementary Fig. 3 ). Full-length tlpB expression seemed to be dispensable for RepG-mediated HP0102 regulation because HP0102::GFP expression was also increased more than two-fold in H. pylori G27 carrying a tlpB mini - hp0102 reporter fusion upon repG deletion. The latter comprises a non-functional 21 codon-long tlpB mini-gene, in which the middle region (544 codons) was deleted (Fig. 2a, b ). Fig. 2: RepG represses HP0102 protein expression through targeting the G-repeat upstream of tlpB-hp0102 . a Schematic representation of translational hp0102 :: gfpmut3 reporter fusion constructs originating from H. pylori strain 26695 (12G) that were integrated into the rdxA locus in H. pylori G27 wildtype and Δ repG . The endogenous tlpB-hp0102 operon in G27 carries a 14G repeat. Red bar: tlpB promoter region; gray: G-repeat upstream of tlpB ; black: tlpB coding region; orange: G- repeat upstream of hp0102 ; dark green: HP0102 coding region; light green: gfpmut3 coding sequence. Arrows indicate the transcriptional start site. b H. pylori G27 WT and Δ repG strains that carry the indicated GFP reporter fusions were grown to exponential phase and HP0102::GFP protein levels were determined by western blot analysis. The relative HP0102::GFP protein levels in the Δ repG mutant (vs. the respective wild-type background) are indicated by bars with corresponding s.d. ( n = 6 biologically independent experiments; corresponding western blot representative is shown in Supplementary Fig. 3 ). ***—highly significant, p -value < 0.001; n.s.—not significant; Student’s t -test, two-tailed. Source data underlying ( b ) is provided as a Source data file. Full size image The hp0102 TTG start codon in the 30-nt-long intergenic region (IGR) between tlpB and hp0102 is preceded by a conserved potential AAGGGT ribosome binding site (RBS) (Fig. 1a and Supplementary Fig. 4b ), suggesting co-transcription but not necessarily co-translation of both genes. A short, variable G-rich sequence (G hp0102 , 3–6G) is found upstream of the hp0102 RBS, which might also be targeted by the C/U-rich loop of RepG sRNA (Supplementary Fig. 4c ). To investigate whether the G hp0102 -repeat is involved in RepG-mediated HP0102 regulation, the 30-nt-long tlpB - hp0102 IGR followed by the hp0102 10 th :: gfpmut3 coding region were fused to the tlpB promoter (P tlpB hp0102 , Fig. 2a ). Equally expressed HP0102::GFP fusion protein levels in the wildtype and the Δ repG mutant carrying the P tlpB hp0102 reporter fusion indicated that the G hp0102 -repeat is not sufficient for RepG-mediated HP0102 expression control (Fig. 2b and Supplementary Fig. 3 ). While slight differences in basal expression levels of HP0102::GFP were observed in the wildtype, neither deletion of the G hp0102 -repeat (ΔG hp0102 ) nor its exchange to an ATTTA-stretch (ATTTA hp0102 ) did significantly affect RepG-mediated repression of HP0102::GFP (Fig. 2b and Supplementary Fig. 3 ). We had previously shown that RepG regulates tlpB expression mainly at the level of translation [21] . Therefore, although harboring a separate RBS, HP0102 expression control through RepG might still be coupled to tlpB mRNA translation. Replacement of the tlpB start codon by a stop codon in the tlpB mini - hp0102 reporter fusion ( tlpB stop - hp0102 , Fig. 2a ) neither affected HP0102::GFP protein expression nor RepG-mediated repression thereof (Fig. 2b and Supplementary Fig. 3 ). This shows that hp0102 translation and regulation is not directly influenced by tlpB translation. Taken together, these data demonstrate that targeting of the homopolymeric G-repeat in the tlpB mRNA leader by the RepG sRNA mediates a coordinated regulation of the tlpB - hp0102 operon, at the transcript and protein level. HP0102 is required for mouse stomach colonization Variable SSRs are often associated with genes important for host-pathogen interactions [18] , [29] . To investigate whether RepG sRNA and/or its targets, tlpB and hp0102 , contribute to virulence and/or survival, we infected mice with either wildtype or non-polar deletion mutant strains of the mouse-adapted strain H. pylori X47-2AL (as in ref. [30] ). While the syntenic organization of the tlpB - hp0102 operon in strain X47-2AL is the same as in strain 26695 (Supplementary Fig. 1c ), the G-repeat in the tlpB mRNA leader is only 7Gs long in X47-2AL compared to 12Gs in 26695 (Supplementary Fig. 4a ). An approximately two-fold repression of tlpB through RepG was observed in strain X47-2AL compared to an about five-fold repression in strain 26695 (Supplementary Fig. 2 ). This is in line with the previously described strain-specific, RepG-mediated tlpB regulation depending on G-repeat length [21] . While no significant change was observed for the Δ repG or Δ tlpB /Δ repG double deletion mutants, in vivo infection studies revealed that the H. pylori X47-2AL Δ tlpB single mutant is slightly attenuated (~1.5-log lower CFU/g of stomach ) in its ability to colonize the murine stomach compared to the wildtype (Fig. 3b ). This minor effect suggests that both RepG and TlpB are largely dispensable for H. pylori mouse stomach colonization. In contrast, no bacteria could be recovered from the stomachs of mice infected with the ∆ tlpB-hp0102 , Δ tlpB - hp0102 /∆ repG , and ∆ hp0102 deletion mutants (Fig. 3b, d ), indicating that hp0102 is essential for H. pylori to colonize mice. Accordingly, stomach colonization was restored in independent infection experiments, in which either the single Δ hp0102 or double Δ tlpB - hp0102 mutants were complemented with either the whole tlpB-hp0102 operon or only hp0102 expressed from the tlpB promoter (P tlpB ) in the rdxA locus (Fig. 3c, d ). A slightly reduced colonization level compared to wildtype (WT) was still observed in the Δ hp0102 + hp0102 strain, which might be due to altered hp0102 expression, e.g., caused by the fusion of the tlpB-hp0102 intergenic region (IGR) to P tlpB . Overall, our in vivo infection studies identified hp0102 as an essential factor for colonization of the murine stomach by H. pylori . Therefore, we aimed to explore a potential link between the variable G-repeat and host colonization that would rely on the function of HP0102. Fig. 3: HP0102 is essential for mice stomach colonization with H. pylori strain X47-2AL. a , c Schematic representation of the construction of H. pylori X47-2AL ∆ repG and ∆ tlpB/hp0102 deletion mutant and complementation strains. TSS are denoted as +1 (black arrows). The repG gene and the tlpB promoter (P tlpB ) are shown in red. The hp0102 gene is shown in green. b , d About 10 8 bacteria of H. pylori X47-2AL WT or indicated mutant strains were orogastrically administered to NMRI Swiss mice. As a control, mice were infected with peptone broth only. Four weeks post infection, mice were sacrificed and colony-forming units (CFUs) per gram of stomach weight were calculated by serial dilutions and plating assays. Each circle indicates the colonization titer in the stomach of a single mouse. The horizontal bars represent the geometric mean for each group of data ( n = 5/4 non-infected control animals for panel b/d, respectively; n = 7 for mice infected with indicated H. pylori strains). ***—highly significant, p -value < 0.001; **—very significant, p -value < 0.01; n.s.—not significant; Mann–Whitney test (Prism), two-tailed. Source data underlying ( b , d ) are provided as a Source data file. Full size image HP0102 is involved in O-chain biosynthesis The HP0102 protein sequence contains several motifs of the glycosyltransferase family 2 (GT-2; www.kegg.jp , http://pfam.sanger.ac.uk/ , http://www.cazy.org/ ), suggesting HP0102 is involved in LPS biosynthesis. While at the time of this study, the precise function of HP0102 was unknown, it was recently described to act as a fucosyltransferase involved in O-chain biosynthesis in H. pylori strain G27 [10] . In line with the study by Li and colleagues [10] , we also observed that H. pylori X47-2AL ∆ hp0102 deletion mutants have only rough-form LPS, i.e. lack the O-chains, and no Lewis x antigens could be detected on western blots (Fig. 4a , lanes 5–6 and 9–10). In contrast, the ∆ repG , ∆ tlpB , and ∆ tlpB /∆ repG mutant strains showed the same smooth LPS profiles (composed of lipid A-core and O-antigens) as wildtype, with comparable Lewis x antigens levels (Fig. 4a , lanes 1–4). Complementation of ∆ tlpB - hp0102 and ∆ hp0102 with either the tlpB - hp0102 operon or with hp0102 alone restored smooth LPS patterns and wild-type Lewis x expression (Fig. 4a , lanes 7–8 and 11). Next, we further validated this function of HP0102 in LPS biosynthesis in the most commonly utilized H. pylori laboratory strains, namely 26695 (Fig. 4b , lanes 1 and 6), J99, and G27 (Supplementary Fig. 5 ). Variations in overall LPS patterns were observed among different WT strains supporting previous reports on strain-specific LPS variations [8] . However, irrespective of the parental strain background, mutants lacking hp0102 express only rough LPS. This confirms a conserved function of HP0102 essential for LPS O-chain biosynthesis and Lewis x antigen display, which is also in agreement with HP0102 homologs universally present in different H. pylori strains [10] . The LPS O-chains contribute to antigenicity and serospecificity of native LPS and play an important role in H. pylori virulence [11] , [31] , [32] . Accordingly, the complete abrogation of mouse colonization by the H. pylori X47-2AL hp0102 mutant strain most probably results from its loss of the LPS O-chains. Fig. 4: The hp0102 gene is required for LPS O-antigen biosynthesis and is regulated by RepG sRNA. The WT and indicated mutant strains of H. pylori strains X47-2AL ( a ) and 26695 ( b ) were grown to exponential growth phase, and RNA and protein samples were analyzed by northern and western blot, respectively. b In 26695, the Δ repG mutant was complemented with wild-type RepG (C RepG ) or mutant sRNAs. SL 2 consists of only the second stem-loop and in ΔCU the tlpB binding site (marked in blue) was replaced by an extra-stable tetraloop [21] . RepG sRNA was detected with CSO-0003 (C/U-rich terminator loop) and JVO-2134 (5’ end). 5S rRNA was used as loading control (JVO-0485). Expression of the chemotaxis receptors TlpA, TlpB, TlpC, and TlpD was analyzed using a polyclonal anti-TlpA22 antiserum. Please note that the Δ hp0102 mutant was loaded/analyzed on the same northern and western blots like the WT and indicated sRNA mutant strains; however, samples were not loaded directly next to each other (indicated by dotted line). a , b LPS samples of the indicated strains were separated on 15% SDS-PAGE gels and either directly visualized by silver staining, or electro-blotted to PVDF membrane and probed with a Lewis x antigen-specific antibody. The results shown are representative of at least three independent experiments. Source data underlying ( a , b ) are provided as a Source data file. Full size image In order to narrow down how HP0102 affects LPS O-chain biosynthesis, we constructed several additional LPS mutants (Supplementary Figs. 6 and 7a ) in H. pylori strains 26695 and X47-2AL and compared their LPS profiles with the ∆ hp0102 mutants. These deletions affected LPS core oligosaccharide (HP1284 [8] ), various parts of the O-antigen (HP1039 [33] ; HP1581 [33] ; HP0159 [34] HP0826 [35] ), lipid A modulation (HP0579-0580 [36] ), or LPS O-chain translocation (HP1206 [33] ). Comparing their LPS profiles and Lewis x/y antigen expression to the patterns of the corresponding ∆ hp0102 mutants showed that the deep rough LPS phenotype of the HP0102 deletion mutant most closely resembled the pattern observed for the HP1039 and HP1581 mutant strains (Supplementary Fig. 7b, c ). In addition, deletions of HP0102, HP1039, HP1581, HP0159, HP0826, and HP1206 resulted in the loss of both Lewis x and y antigens. These observations were consistent in both H. pylori strain backgrounds. These mutational analyses together with a previously missing enzyme for the conserved trisaccharide of the O-antigen (previously referred to as the outer core) [8] , indicated HP0102 is involved in the biosynthesis of the trio (Supplementary Fig. 7 ). Indeed, and in line with our observations, Li and colleagues revealed HP0102 as the fucosyltransferase of the LPS trisaccharide using mass spectrometry-based structural LPS analyses [10] . Because both, X47-2AL and 26695, showed stronger signals for Lewis x than Lewis y, all following experiments regarding LPS profiling and Lewis antigen expression were focused on western blot analyses of Lewis x. RepG regulates tlpB-hp0102 and consequently LPS biosynthesis To investigate whether RepG sRNA regulates expression of hp0102 (in addition to tlpB ) and in turn LPS biosynthesis, we examined LPS patterns and Lewis x antigen display in H. pylori strain 26695, in which tlpB is more strongly regulated by RepG than in strain X47-2AL (Supplementary Fig. 2 ). Deletion of repG resulted in increased band intensities in smooth LPS and Lewis x antigen levels in strain 26695 (Fig. 4b , lanes 1–2), indicating regulation of hp0102 by RepG. Complementation of the Δ repG mutant with wild-type (C RepG ) or a mutant RepG sRNA expressing only the second stem-loop with the C/U-rich tlpB binding site (SL2) restored wild-type LPS and Lewis x (Fig. 4b , lanes 3–4). In contrast, deletion of the previously identified C/U-rich tlpB interaction site in RepG (∆CU) [21] , led to increased O-antigen and Lewis x similar as observed for the repG deletion mutant (Fig. 4b , lane 5). These RepG mutant analyses demonstrate that the C/U-rich terminator loop of RepG is sufficient to repress both tlpB and hp0102 . The G-repeat in the tlpB-hp0102 leader determines LPS production While RepG is highly conserved, the length of its G-repeat target in the tlpB leader varies among H. pylori isolates, resulting in strain-specific tlpB regulation [21] . RepG represses TlpB protein expression in H. pylori strains X47-2AL (7G, two-fold; Fig. 4a ) and 26695 (12G, five-fold; Fig. 4b ). In contrast, TlpB protein levels were unaffected or increased upon repG deletion in strains J99 (13G) and G27 (14G, two-fold), respectively (Supplementary Fig. 5 ). Deletion of repG did not significantly affect LPS profiles in strains X47-2AL, J99, and G27 (Fig. 4a , lane 2 and Supplementary Fig. 5 ), but resulted in increased band intensities in smooth LPS and Lewis x antigen levels in strain 26695 (Fig. 4b , lanes 1–2), confirming a strain-specific G-repeat-dependent tlpB-hp0102 regulation. To more systematically investigate whether the G-repeat length impacts RepG-mediated control of hp0102 , the G-repeat was either deleted (ΔG) or mutated from 6 to 16 guanines (6–16G) in the tlpB mRNA leader of H. pylori 26695 expressing TlpB::3xFLAG (as in ref. [21] ). RT-qPCR analysis of tlpB and hp0102 mRNA levels in the tlpB leader variants (∆G, 6–16G) of H. pylori 26695 revealed that expression of both genes is indeed dependent on the G-repeat length (Fig. 5a , left panel). While deletion of the G-repeat (ΔG) had only a minor influence on tlpB and hp0102 mRNA levels when compared to wildtype (12G), expression of both genes was increased in the 6G-variant. A gradual decrease in tlpB and hp0102 mRNA levels was observed with an increasing number of guanines in the tlpB mRNA leader, reaching a minimum level for 8–12Gs. Further extension of the G-stretch from 13–16Gs resulted again in elevated transcript abundances. Whereas deletion of repG affected neither tlpB nor hp0102 expression in ∆G, 6G, and 13–16G, significantly increased mRNA levels were observed in the 7–12G leader mutants upon repG deletion (Fig. 5a , right panel). Fig. 5: The G-repeat length impacts RepG-mediated tlpB - hp0102 co-regulation and in turn smooth LPS production. a (Left panel) RT-qPCR of relative tlpB and hp0102 mRNA levels of different tlpB leader mutants (ΔG, 6–16G) in the H. pylori 26695 wild-type background. The mRNA level of each gene in the tlpB 6G-leader mutant was used as reference and set to 1. (Right panel) Relative fold changes of tlpB and hp0102 mRNA levels upon repG deletion in H. pylori 26695 tlpB leader mutants when compared to the respective wild-type backgrounds. The fold changes are shown as mean of three biological replicates with corresponding error bars (s.d.). ***—highly significant, p -value < 0.001; **—very significant, p -value < 0.01; *—significant, p -value < 0.05; n.s.—not significant; Student’s t -test, two-tailed. b The LPS patterns and Lewis x antigen levels of tlpB leader mutants in H. pylori 26695 wild-type and ∆ repG mutant backgrounds were analyzed by silver staining and western blot analysis with anti-Lewis x antigen antibody, respectively. Expression of the chemotaxis receptors was analyzed by an anti-TlpA22 antiserum. Note that tlpB leader mutants express FLAG-tagged TlpB [21] . A representative silver-stained PAA-gel and western blot are shown (out of three independent experiments). Source data underlying ( a , b ) are provided as a Source data file. Full size image Next, we investigated whether SSR-dependent regulation of the tlpB-hp0102 operon also affects LPS biosynthesis. Every tlpB mRNA leader variant (∆G, 6–16G) of the wild-type background expresses smooth LPS. However, similar to gradual TlpB expression levels depending on the G-repeat length, varying O-chain and Lewis x profiles were detected (Fig. 5b , lanes 1–12). Whereas tlpB leader length variants of 6–8G and 13–16G displayed increased expression levels, decreased amounts of O-chains and Lewis x levels were detected for 9–11G variants in comparison to WT (12G; Fig. 5b and Supplementary Fig. 8 ). The gradual TlpB and LPS/Lewis x patterns were lost upon repG deletion, confirming that the G-repeat length indeed affects sRNA-mediated regulation. The strongest effects were observed in tlpB mRNA leader mutants that comprise a G-repeat of 9–12Gs, in which deletion of repG resulted in significantly increased O-chain and Lewis x levels. In contrast, LPS patterns remained almost unaltered in the ∆G, 6–8G, and 13–16G variants. In conclusion, the amounts of Lewis x antigen and TlpB protein levels closely correlate in the varying G-repeat strains. RepG significantly represses TlpB protein and smooth LPS biosynthesis/O-antigen levels in tlpB leader variants that comprise a 9–12G-long repeat, in line with the previously defined optimal window for RepG-mediated repression [21] . Overall, these data show that the length of the G-repeat in the tlpB mRNA leader impacts RepG-mediated co-regulation of tlpB and hp010 2 and consequently, smooth LPS production. Deletion of hp0102 leads to reduced growth upon salt stress LPS is essential for the integrity and functionality of the bacterial outer membrane and protects the bacteria against surface stress [37] . For example, divalent cation bridging of phosphates on lipid A and/or the core oligosaccharide of LPS contributes to the stabilization of the outer membrane and ensures its function as an effective permeability barrier. Bacteria with incomplete LPS, e.g., rough LPS, are more sensitive to environmental stresses, including osmotic stress [38] . To examine whether, or to which extent, the hp0102 -dependent rough LPS phenotype affects H. pylori survival under osmotic stress, the growth of the wildtype and mutant strains of H. pylori X47-2AL, 26695, J99, and G27 was examined under elevated sodium chloride (NaCl) concentrations, an often-used method to simulate osmotic stress conditions. A drastic decrease in viable bacterial counts was observed on high-salt plates for all tested H. pylori mutants lacking hp0102 (Fig. 6a and Supplementary Fig. 9a ). Hence, HP0102-dependent smooth LPS production is required to maintain the integrity of the H. pylori cell envelope. Complementation of the H. pylori X47-2AL Δ hp0102 mutant only partially restored wild-type growth (Fig. 6a ), which might be due to a slightly different expression of HP0102 in the complementation strain. In line with hp0102 being repressed by RepG in H. pylori strain 26695, deletion of repG rendered H. pylori more resistant to high-salt conditions (Fig. 6a ). In contrast, an increased sensitivity toward osmotic stress was observed for the H. pylori G27 Δ repG mutant (Supplementary Fig. 9a ). Because smooth LPS biosynthesis seems to be unaffected by RepG in G27 (Supplementary Fig. 5 ), this phenotype might be linked to the regulation of other, so far undefined, targets of RepG. Fig. 6: RepG affects sensitivity to salt stress and polymyxin B via regulation of hp0102 . a H. pylori X47-2AL and 26695 WT and indicated mutant strains were grown in liquid culture to exponential growth phase (OD 600 of 1). Indicated ten-fold dilutions of the bacterial suspensions were spotted on GC-agar plates containing 80 mM (basal concentration), 200 mM (mild stress), or 260 mM (harsh stress) sodium chloride. Plates were incubated for 3–5 days at 37 °C under microaerobic conditions. The results shown are representative of at least two independent experiments. b Polymyxin B sensitivity testing for H. pylori X47 and 26695 WT and indicated mutant strains using E-tests. Error bars indicate s.d. for n = 3 independent biological experiments. ****— highly significant, p -value < 0.0001; **—very significant, p -value < 0.01; n.s.—not significant; Student’s t -test, two-tailed. c (Upper panel) Polymyxin B MICs of H. pylori 26695 tlpB mRNA leader variants in the wild-type background. (Lower panel) Relative fold changes in polymyxin B sensitivity (MICs) upon repG deletion in different tlpB leader variants when compared to the respective wild-type backgrounds ( n = 2 for WT/∆ repG _∆G, ∆ repG _6G, WT/∆ repG _7-9G, WT/∆ repG _11G, WT/∆ repG _13G, WT/∆ repG _15-16G; n = 3 for WT_6G, WT/∆ repG _10G, WT/∆ repG _12G, WT/∆ repG _14G). d Model of RepG-mediated regulation of TlpB and HP0102. The genes encoding the chemotaxis receptor TlpB (dark gray) and the fucosyltransferase HP0102 (green) are transcribed as a bicistronic mRNA and play a role in chemotaxis [25] and smooth LPS biosynthesis (light green) as well as protection against membrane stress (indicated by red arrow), respectively. Deletion of hp0102 leads to loss of O-antigens and a rough LPS phenotype (dark green). Antisense base-pairing of the C/U-rich terminator loop of RepG sRNA to the homopolymeric G-repeat in the 5′ UTR of the tlpB-hp0102 mRNA results in post-transcriptional co-regulation of tlpB and hp0102 at the transcript and protein level. Depending on the G-repeat length, RepG mediates both repression (7–12Gs) and activation (≥14Gs) of tlpB and hp0102 . OM/IM—outer/inner membrane, RBS—ribosome binding site, AUG/UUG—start codons, UAA—stop codon. Source data underlying ( b , c ) are provided as a Source data file. Full size image RepG affects polymyxin B sensitivity by repression of hp0102 Modifications in the LPS structure have been shown to affect H. pylori resistance to cationic antimicrobial peptides (CAMPs [9] , [12] ), which represent critical components of the human innate immune system. CAMPs interact with negatively charged phospholipid groups or the LPS lipid A anchor, inducing bacterial lysis and cell death. Using E-test strips, we measured the resistance of H. pylori X47-2AL, 26695, J99, and G27 wildtype and chosen mutant strains to polymyxin B (PxB), a membrane-targeting antibiotic and surrogate for host CAMPs. Irrespective of the parental strain background, Δ hp0102 mutants displayed reduced minimal inhibitory concentrations (MICs) to PxB compared to WT (Fig. 6b and Supplementary Fig. 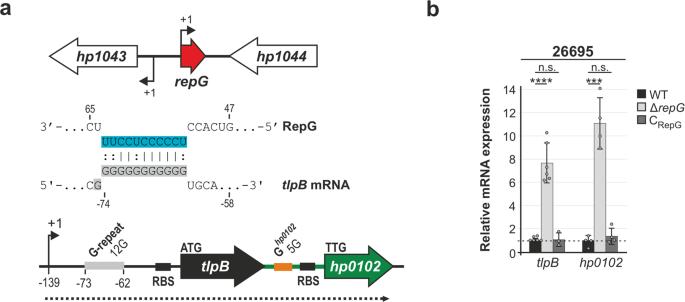Fig. 1: RepG sRNA represses expression of thetlpB-hp0102mRNA. aInH. pyloristrain 26695, RepG sRNA is transcribed from the intergenic region betweenhp1043andhp1044, encoding an orphan response regulator and a protein of unknown function. The C/U-rich terminator loop of RepG (blue) binds to a homopolymeric G-repeat (12G, light gray) in the 5′ UTR of the bicistronictlpB-hp0102mRNA (dotted line), encoding a chemotaxis receptor and a protein of unknown function21. Transcriptional start sites (TSS, +1; ref.28) and ribosome binding sites (RBS) are indicated by arrows and black bars, respectively. Numbers designate the distance to thetlpBstart codon. A G-rich sequence (Ghp0102, orange) was identified in thetlpB-hp0102IGR.bRT-qPCR analysis of RepG-dependent regulation oftlpBandhp0102inH. pyloristrain 26695 wildtype (WT),repGdeletion (∆repG), and complementation (CRepG) mutants. Wild-type mRNA levels of each gene were set to 1, and relative mRNA levels in mutants are shown as bars. Values are shown as mean ± standard deviations (s.d.) forn= 6 (tlpB; exception CRepGn= 3) andn= 4 (hp0102) biologically independent experiments. ****—highly significant,p-value < 0.0001; ***—highly significant,p-value < 0.001; n.s.—not significant; Student’st-test, two-tailed. Source data underlying (b) is provided as a Source data file. 9b–d , Supplementary Table 1 ). Complementation of Δ hp0102 in X47-2AL restored wild-type PxB susceptibility, suggesting that the alteration of the LPS structure through hp0102 is associated with antibiotic sensitivity in H. pylori . While no significant effect was observed upon repG deletion in X47-2AL, J99, and G27, the 26695 Δ repG mutant was twice as resistant to PxB as the wildtype. Deletion of tlpB in X47-2AL leads to a negligible reduction in MIC and a non-significant increase in strain 26695. Thus, the observed effects on PxB sensitivity seem to be mediated primarily by modulation of hp0102 expression (Fig. 6b , Supplementary Table 1 ). Moreover, deletion of hp0102 affects PxB sensitivity more strongly compared to mutants defective in O-chain length (HP0826 and HP0159) but less pronounced when compared to deletion mutants completely devoid of O-chain (HP1039 and HP1581), the core oligosaccharide (HP1284), and lipid A (HP0579/80) (Supplementary Fig. 9c, d and Supplementary Table 1 ). This additionally supports the recently reported function of HP0102 as the LPS trisaccharide fucosyltransferase [10] . Next, we characterized PxB sensitivity of tlpB-hp0102 G-repeat leader variants of 26695 WT and Δ repG . While sensitivity to PxB was not affected in ΔG, the 6–8G and 13–16G variants were more resistant to PxB than the wildtype (12G; Fig. 6c , upper panel). Consistent with reduced smooth LPS expression (Fig. 5b ), 9–11G mutants were more susceptible to PxB. In the ∆ repG background, all tlpB mRNA leader variants displayed similar MICs (data not shown). Accordingly, deletion of repG resulted in two- to four-fold increased resistance to PxB for tlpB leader variants 9–12G (Fig. 6c , lower panel), whereas MICs remained unaltered in almost all other leader mutants. Taken together, these data demonstrate that RepG-mediated expression control of hp0102 leads to gradual control of LPS O-chain synthesis and thereby contributes to the integrity and permeability of the bacterial membrane and H. pylori susceptibility to PxB. Here, we showed that the H. pylori HP0102 protein is involved in LPS O-chain production, essential for murine stomach colonization and important for resistance to the membrane-targeting antibiotic PxB. Moreover, we demonstrated that hp0102 is post-transcriptionally regulated by RepG sRNA through base-pairing to a variable, homopolymeric G-repeat in the 5′ UTR of the bicistronic tlpB-hp0102 mRNA. In contrast to SSR-based phase-variable ON/OFF gene expression switches, this unique mode of regulation allows for a fine-tuned control of hp0102 and in turn smooth LPS biosynthesis, which might be required for H. pylori adaptation to different host niches. Binding of RepG to the G-repeat upstream of the tlpB open reading frame is sufficient to regulate tlpB and hp0102 both at the transcript and protein level (Fig. 2 ). Our GFP reporter assay showed that hp0102 translation is likely independent of tlpB , suggesting that RepG-mediated repression of hp0102 is rather based on ribosomal recruitment and/or destabilization of the entire mRNA than on direct translational coupling. RepG regulates tlpB expression at the translational level and induces structural rearrangements within the tlpB mRNA when binding to the G-repeat [21] . Sequestration of the G-repeat, which is located relatively far upstream of the RBS and might function as a translational enhancer and/or ribosome standby site, could affect both tlpB and hp0102 translation similarly as previously shown for other sRNAs [39] , [40] . Furthermore, structural rearrangements caused by RepG binding might also lead to the inhibition of translation elongation and/or whole transcript destabilization by RNase recruitment [41] . Bacterial adaptive changes, including modulation of LPS synthesis and structure, play an important role during infection. In our study, we observed H. pylori Δ hp0102 mutants display rough LPS phenotypes, indicative of O-antigen loss, supporting its recent identification as the trisaccharide fucosyltransferase [10] . H. pylori LPS can mimic host structures and is essential for resistance to host-derived CAMPs [6] , making it a key surface determinant required for colonization and persistence as shown in rodent models [12] , [31] , [32] . In line with a previous transposon mutagenesis screen in strain G27, which indicated hp0102 is a candidate gene required for colonization in mice [42] , we observed that mice stomach colonization of an H. pylori X47-2AL ∆ hp0102 mutant is completely abolished. Similarly, other H. pylori glycosyltransferases involved in LPS biosynthesis are also essential for colonization of mice [8] , [43] . As LPS core and variable Lewis antigens facilitate immune escape [11] , [44] and promote adherence to the gastric epithelium [45] , [46] , [47] , the Δ hp0102 colonization defect might be associated with an enhanced susceptibility of this mutant to the inflammatory host response and membrane stress within the host and/or its impaired ability to bind to the gastric epithelium. Other functions might also be affected in the H. pylori ∆ hp0102 mutant, such as a recently reported modulation of the expression of the major virulence factor CagA as well as H. pylori chemotaxis [48] . While chemotaxis in H. pylori is important for proper bacterial orientation and localization in the gastric glands [25] , [49] , the X47-2AL ∆ tlpB mutant presented only a mildly reduced murine stomach colonization (Fig. 3 ) and no defect during competitive co-infection experiments [26] , [27] . Together with our data, this indicates that the TlpB chemotaxis receptor is not necessarily required for bacterial growth in the rodent stomach. Further studies are required to evaluate the importance of the tlpB-hp0102 operon co-regulation and its functional implications for H. pylori persistence. Diverse pathogens benefit from SSR-mediated phase variation of surface structures as these allow them to rapidly adapt to changes in their host environment [50] , [51] . 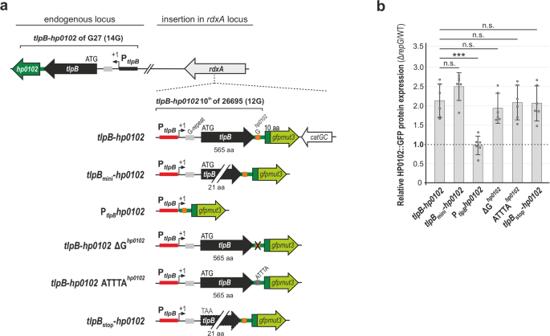Fig. 2: RepG represses HP0102 protein expression through targeting the G-repeat upstream oftlpB-hp0102. aSchematic representation of translationalhp0102::gfpmut3reporter fusion constructs originating fromH. pyloristrain 26695 (12G) that were integrated into therdxAlocus inH. pyloriG27 wildtype and ΔrepG. The endogenoustlpB-hp0102operon in G27 carries a 14G repeat. Red bar:tlpBpromoter region; gray: G-repeat upstream oftlpB; black:tlpBcoding region; orange: G-repeatupstream ofhp0102; dark green: HP0102 coding region; light green:gfpmut3coding sequence. Arrows indicate the transcriptional start site.bH. pyloriG27 WT and ΔrepGstrains that carry the indicated GFP reporter fusions were grown to exponential phase and HP0102::GFP protein levels were determined by western blot analysis. The relative HP0102::GFP protein levels in the ΔrepGmutant (vs. the respective wild-type background) are indicated by bars with corresponding s.d. (n= 6 biologically independent experiments; corresponding western blot representative is shown in Supplementary Fig.3). ***—highly significant,p-value < 0.001; n.s.—not significant; Student’st-test, two-tailed. Source data underlying (b) is provided as a Source data file. The H. pylori genome contains variable SSRs in a number of outer membrane proteins, adhesins, or LPS-biosynthetic or -modifying enzymes (Supplementary Table 2 ) [52] , [53] . 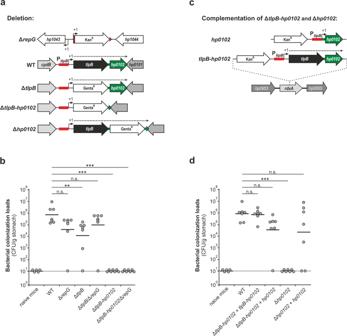Fig. 3: HP0102 is essential for mice stomach colonization withH. pyloristrain X47-2AL. a,cSchematic representation of the construction ofH. pyloriX47-2AL ∆repGand ∆tlpB/hp0102deletion mutant and complementation strains. TSS are denoted as +1 (black arrows). TherepGgene and thetlpBpromoter (PtlpB) are shown in red. Thehp0102gene is shown in green.b,dAbout 108bacteria ofH. pyloriX47-2AL WT or indicated mutant strains were orogastrically administered to NMRI Swiss mice. As a control, mice were infected with peptone broth only. Four weeks post infection, mice were sacrificed and colony-forming units (CFUs) per gram of stomach weight were calculated by serial dilutions and plating assays. Each circle indicates the colonization titer in the stomach of a single mouse. The horizontal bars represent the geometric mean for each group of data (n= 5/4 non-infected control animals for panel b/d, respectively;n= 7 for mice infected with indicatedH. pyloristrains). ***—highly significant,p-value < 0.001; **—very significant,p-value < 0.01; n.s.—not significant; Mann–Whitney test (Prism), two-tailed. Source data underlying (b,d) are provided as a Source data file. When sequentially isolated from human patients [54] , [55] , [56] , [57] , [58] or re-isolated from animal colonization experiments [59] , [60] , even H. pylori strains within the same host exhibited varying G-repeat length in the tlpB 5′ UTR (Supplementary Table 3 ). This suggests that tlpB-hp0102 is associated with a phase-variable SSR. So far, Lewis antigen-producing fucosyltransferases have been described to be controlled by SSRs in an ON/OFF manner [14] , [15] , [16] , [60] , [61] , [62] . In contrast, we uncovered a gradual regulation of an operon encoding two proteins important for H. pylori colonization, namely the chemotaxis receptor TlpB and HP0102 required for O-chain display, by a sRNA that targets a SSR in the mRNA leader sequence, resulting in gradual changes of smooth LPS. This “LPS fine-tuning” might help H. pylori to balance the fine line between host immune evasion and lack of sufficient adherence potential [63] , [64] , [65] . The here described gradual display of LPS O-chain might increase heterogeneity in the population, enabling H. pylori to adapt and survive in the gastric mucosa of individual host niches and thus contributing to persistence. HP0102-mediated structural LPS changes can support this adaptation as demonstrated by an increased sensitivity of a hp0102 mutant to high salt concentrations and to membrane-targeting antibiotics such as PxB, which is a surrogate of host-derived CAMPs. The regulation of hp0102 by the RepG sRNA thereby adds to a number of bacterial sRNAs that impact antibiotic resistance, e.g., by regulating expression of drug transporters or efflux proteins, biofilm formation, or metabolic enzymes involved in cell envelope synthesis or LPS biosynthesis [66] . The RepG-dependent regulatory mechanism presents several unique features. We demonstrated that the G-repeat length mediates repression (7–12Gs) or activation (≥14Gs) of the tlpB - hp0102 operon by RepG. This is a unique regulatory mechanism linking post-transcriptional gene expression control to phase variation. To the best of our knowledge, intergenic SSRs that affect full-length LPS O-chain display in a reversible and rheostat-like fashion at the post-transcriptional level, as described in this study, have not been identified in other bacterial pathogens so far. Besides hp0102 , three other LPS-modifying enzymes are associated with intergenic SSRs in H. pylori strain 26695 (Supplementary Table 2 ). Whether these intergenic SSRs affect promoter strength and/or are targeting sites for sRNAs still needs to be examined. At the transcriptional level, for example, length variation of a promoter-associated, intergenic SSR has been described to result in low, mediate, and high expression levels of the major H. pylori adhesin SabA [67] . Future experiments are needed to evaluate if the presence or expression of RepG sRNA itself might provide a selective force toward a certain length of the G-repeat, thereby influencing the rate of SSR polymorphism. Phase variation is usually stochastic and random; however, gene regulation has been shown to be integrated with phase variation events. For example, phase variation of methyltransferases can modulate bacterial gene expression via epigenetic mechanisms [68] and Dam methylation can impact phase-variable ON/OFF switching [69] . Moreover, sRNA-mediated regulation of the P-fimbriae phase regulator papI affects the ON/OFF switch and, thus, expression of P-fimbriae on the surface of uropathogenic E. coli [70] . And transcription of a cis -encoded sRNA antisense to the pilE promoter impacts pilin antigenic variation in Neisseria meningitidis [71] . Recently, we and others also uncovered that sRNAs themselves can be associated with SSRs and identified a phase-variable sRNA, NikS, that acts as a global post-transcriptional regulator of the major virulence genes of H. pylori [72] , [73] . In H. pylori , alterations in the LPS structure of H. pylori have been described at low pH [74] . The post-transcriptional regulation of the tlpB-hp0102 operon through RepG might provide an additional layer of LPS gene expression control under varying environmental conditions. As antisense transcription has been identified to various genes involved in H. pylori LPS biosynthesis [28] , regulation of surface structures by cis- or trans -encoded antisense RNAs might be a more general theme in H. pylori gene expression control. In conclusion, our study has unraveled a rheostat-like type of phase variation-dependent, post-transcriptional regulation of surface structures that are important for the colonization capacity of a bacterial pathogen. 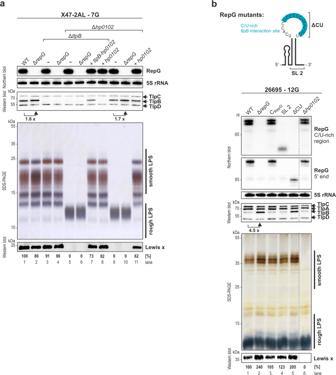Fig. 4: Thehp0102gene is required for LPS O-antigen biosynthesis and is regulated by RepG sRNA. The WT and indicated mutant strains ofH. pyloristrains X47-2AL (a) and 26695 (b) were grown to exponential growth phase, and RNA and protein samples were analyzed by northern and western blot, respectively.bIn 26695, the ΔrepGmutant was complemented with wild-type RepG (CRepG) or mutant sRNAs. SL 2 consists of only the second stem-loop and in ΔCU thetlpBbinding site (marked in blue) was replaced by an extra-stable tetraloop21. RepG sRNA was detected with CSO-0003 (C/U-rich terminator loop) and JVO-2134 (5’ end). 5S rRNA was used as loading control (JVO-0485). Expression of the chemotaxis receptors TlpA, TlpB, TlpC, and TlpD was analyzed using a polyclonal anti-TlpA22 antiserum. Please note that the Δhp0102mutant was loaded/analyzed on the same northern and western blots like the WT and indicated sRNA mutant strains; however, samples were not loaded directly next to each other (indicated by dotted line).a,bLPS samples of the indicated strains were separated on 15% SDS-PAGE gels and either directly visualized by silver staining, or electro-blotted to PVDF membrane and probed with a Lewis x antigen-specific antibody. The results shown are representative of at least three independent experiments. Source data underlying (a,b) are provided as a Source data file. Bacterial strains, oligonucleotides, and plasmids Helicobacter pylori and Escherichia coli strains are listed in Supplementary Table 4 . DNA oligonucleotides and plasmids are summarized in Supplementary Tables 5 and 6 , respectively. Sequence information on 5′ UTRs or coding sequences of tlpB and hp0102 used in the GFP-reporter assays and tlpB leader variants are shown in Supplementary Tables 7 and 8 , respectively. Bacterial growth E. coli strains were grown in Luria Bertani (LB) medium supplemented with 100 µg/ml ampicillin, 20 µg/ml chloramphenicol, 20 µg/ml kanamycin, and/or 10 µg/ml gentamicin if applicable. H. pylori strains were grown on GC-agar (Oxoid) plates supplemented with 10% horse serum (DHS, Biochrom AG), 1% vitamin mix, 10 µg/ml vancomycin, 5 µg/ml trimethoprim, and 1 µg/ml nystatin. For transformant selection and growth of mutant strains, 20 µg/ml kanamycin, 20 µg/ml chloramphenicol, 10 µg/ml gentamicin or 10 µg/ml erythromycin were added. For liquid cultures, 15 or 50 ml Brain Heart Infusion medium (BHI, Roth) supplemented with 10% FBS (Biochrom AG) and 10 µg/ml vancomycin, 5 µg/ml trimethoprim, and 1 µg/ml nystatin were inoculated with H. pylori strains from plates to a final OD 600 of 0.02–0.04 and grown under agitation at 140 rpm in 25 cm 3 or 75 cm 3 cell culture flasks. Bacteria were grown at 37 °C in a HERAcell 150i incubator (Thermo Scientific) in a microaerobic environment (10% CO 2 , 5% O 2 , and 85% N 2 ). Construction of Helicobacter pylori mutant strains All mutant strains are listed in Supplementary Table 4 . Mutants were constructed by homologous recombination and natural transformation of PCR-amplified constructs carrying either the aphA- 3 kanamycin [75] , the catGC chloramphenicol [76] , the aac (3)-IV apramycin/gentamicin [77] or rpsL-erm erythromycin [78] resistance cassette flanked by ~500 bp homology regions up- and downstream of the respective genomic locus. Briefly, H. pylori was grown from frozen stocks, passaged twice, then streaked on a fresh GC-agar plate and grown for 6–8 h at 37 °C under microaerobic conditions. For transformation, 500 ng up to 1 µg purified PCR product was added to the cells. After incubation for 14–16 h at 37 °C, cells were re-streaked on selective plates with the corresponding antibiotic. Genomic DNA (gDNA) of mutants was isolated using NucleoSpin Plasmid Kit according to the manufacturer’s instructions and mutants were checked by PCR and sequencing. The H. pylori 26695 sRNA mutant (Δ repG , C RepG , SL 2, ΔCU) as well as Δ tlpB deletion strains, and tlpB mRNA leader variants (ΔG, 6–16G in wild-type and Δ repG mutant strain backgrounds), and the repG deletion mutants in diverse H. pylori strains (G27 and J99) were constructed in our previous study [21] . Construction of X47-2AL mutant strains for mouse infections To delete repG in the mouse-adapted H. pylori strain X47-2AL, a Δ repG deletion construct ( aphA -3 flanked by 500 nt up- and downstream of repG ) was amplified by PCR using JVO-5070/-5072 and gDNA from JVS-7014 ( H. pylori 26695 Δ repG , ref. [28] ). The purified PCR product was transformed into CSS-0996 ( H. pylori X47-2AL wildtype). Deletion of repG was verified by PCR using JVO-5069/-5257 on gDNA, resulting in strain CSS-0997 (X47-2AL Δ repG ). The tlpB gene was deleted from strain CSS-0996 ( H. pylori X47-2AL wildtype) by insertion of the aac (3)-IV cassette. To avoid potential polar effects of Δ tlpB on the expression of the downstream gene hp0102 , the tlpB coding region was replaced by a non-polar gentamicin resistance cassette ( aac (3)-IV), leaving the tlpB promoter and 5′ UTR intact. Therefore, a plasmid containing the aac (3)-IV cassette flanked by 500 nt up- and downstream of the H. pylori strain X47-2AL tlpB locus was cloned into E. coli . 500 nt up- and downstream of the tlpB open reading frame were amplified from gDNA of strain CSS-0996 ( H. pylori X47-2AL wildtype) using CSO-0039/-0040. The resulting PCR product was Xba I/ Xho I digested and introduced into likewise digested pJV752-1. Next, the resulting plasmid (pBA5-4) was used as a template for a PCR with CSO-0942/-1745 to replace the aac (3)-IV cassette with the tlpB open reading frame using an Eco RI restriction site. In parallel, a PCR with phosphorylated CSO-0263 and CSO-0293 on pUC1813apra [77] was performed and the resulting PCR product was digested with Eco RI. Both Eco RI - digested PCR products (plasmid with tlpB up- and downstream region as well as aac (3)-IV) were ligated and transformed into E. coli . Insertion of the aac (3)-IV cassette was verified by colony PCR (pZE-A/CSO-0293), resulting in pBA13-5. A PCR product amplified with CSO-0039/-0040 from pSP13-5 was transformed into H. pylori X47-2AL (CSS-0996). Positive gentamicin-resistant mutants were confirmed by PCR on gDNA using CSO-0051/-0293, resulting in strain CSS-1123 (X47-2AL Δ tlpB ). An analogous cloning strategy was used for the construction of the tlpB - hp0102 double deletion mutant (Δ tlpB - hp0102 ) and deletion of hp0102 alone (Δ hp0102 ). Please note that in these mutants, the aac (3)-IV cassette was inserted 77 nt upstream of the hp0102 stop codon to avoid interference with hp0101 expression. For deletion of the entire tlpB - hp0102 operon, a PCR-fragment containing 500 nt downstream of the H. pylori X47-2AL hp0102 open reading frame (CSO-0871/-1359 on gDNA of CSS-0996) was inserted into pBA13-5 (CSO-0874/0293 on pBA13-5) using oligo-introduced Eco RI/ Xho I restriction sites. The ligated PCR-products were transformed into E. coli , resulting in pSP127-3. Insertion of the 500 nt downstream of hp0102 was verified by colony PCR using pZE-A/CSO-1359. The tlpB (500up)- aac (3)-IV- hp0102 (500down) deletion construct was amplified from pSP127-3 with CSO-0040/-1359 and transformed into H. pylori X47-2AL (CSS-0996). Positive gentamicin-resistant mutants were confirmed by PCR on gDNA using CSO-0051/-0293, resulting in strain CSS-1743 (X47-2AL Δ tlpB - hp0102 ). In order to delete hp0102 alone, a PCR-product containing 500 nt upstream of the hp0102 open reading frame was amplified using CSO-1737/-1739 on gDNA of CSS-0996. This PCR product was Xba I /Bam HI digested and ligated together with a likewise digested PCR-product amplified from pSP127-3 using CSO-0873/3195. The resulting plasmid pSP186-2 was checked by PCR using pZE-A and CSO-1739. A PCR product ( hp0102 (500up)- aac (3)-IV- hp0102 (500down)) amplified from pSP186-2 with CSO-1737/-1359 was transformed into H. pylori X47-2AL wildtype (CSS-0996). Positive gentamicin-resistant mutants were confirmed by PCR on gDNA (CSO-1738/0293), resulting in CSS-2019 (X47-2AL Δ hp0102 ). For construction of double deletion mutants Δ tlpB /Δ repG , Δ tlpB - hp0102 /Δ repG, and Δ hp0102 /Δ repG , the sRNA deletion construct ( aphA -3 flanked by 500 nt up- and downstream of repG ) amplified by PCR using JVO-5070/-5072 on gDNA from JVS-7014 ( H. pylori 26695 Δ repG ) was transformed into CSS-1123 (X47-2AL Δ tlpB ), CSS-1743 (X47-2AL Δ tlpB - hp0102 ), and CSS-2019 (X47-2AL Δ hp0102 ). The double deletion strains CSS-1769 (X47-2AL Δ tlpB /Δ repG ), CSS-1773 (X47-2AL Δ tlpB - hp0102 /Δ repG ) and CSS-2022 (X47-2AL Δ hp0102 /Δ repG ) were verified by PCR using JVO-5069/-5257. The Δ tlpB - hp0102 and Δ hp0102 deletion mutants were complemented with either the entire tlpB - hp0102 operon or hp0102 alone in the unrelated rdxA locus. Therefore, plasmids containing rdxA (500up)- aphA -3- tlpB - hp0102 - rdxA (500down) or rdxA (500up)- aphA -3-P tlpB hp010 2- rdxA (500down) were constructed in E. coli . First, Cla I/ Nde I-digested PCR products amplified with CSO-1740/-1741 on gDNA of CSS-0996 ( H. pylori X47-2AL) and CSO-0146/-0147 on pBA4-2 (pSP39-3 carrying aac (3)-IV gentamicin resistance cassette) were ligated and transformed into E. coli , resulting in pSP189-4. The aac (3)-IV gentamicin resistance cassette from pSP189-4 was exchanged with the aphA -3 kanamycin resistance cassette by ligation of Bam HI/ Nhe I - digested PCR products amplified with CSO-0940/-0941 on pSP189-4 and CSO-1813/-1814 on gDNA of JVS-7014 ( H. pylori 26695 Δ repG ). The resulting plasmid pSP190-1 ( rdxA (500up)- aphA -3- tlpB - hp0102 - rdxA (500down)) was used as template for cycle-PCR using CSO-1743/-1742. This PCR product was Dpn I-digested and directly transformed into E. coli , resulting in pSP192-1 ( rdxA (500up)- aphA -3-P tlpB hp0102 - rdxA (500down)). PCR products amplified by CSO-0017/-0018 on pSP190-1 and pSP192-1 were used for transformation in CSS-1743 (X47-2AL Δ tlpB - hp0102 ) and CSS-2019 (X47-2AL Δ hp0102 ). The obtained, kanamycin-resistant strains CSS-2046 (X47-2AL Δ tlpB - hp0102 + tlpB - hp0102 ), CSS-2080 (X47-2AL Δ tlpB - hp0102 + hp0102 ), and CSS-2087 (X47-2AL Δ hp0102 + hp0102 ) were verified by PCR using oligos CSO-0207/-1813 and sequencing by CSO-0206/-0086. Construction of Δ hp0102 in H. pylori 26695, G27, and J99 The hp0102 gene was deleted from strain CSS-0004 ( H. pylori 26695 wildtype), CSS-0010 ( H. pylori G27 wildtype) and CSS-0001 ( H. pylori J99 wildtype) by insertion of the rpsL-erm cassette, which confers dominant streptomycin susceptibility and erythromycin resistance [78] . A plasmid containing the rpsL-erm cassette flanked by 500 nt up- and downstream of the hp0102 open reading frame was generated in E. coli . A PCR product corresponding to 500 nt upstream of hp0102 (CSO-0869/-0870 on gDNA of CSS-0004) was Bam HI/ Xho I-digested and ligated into likewise digested pSP60-2 [21] , resulting on pBA1-1. About 500 nt downstream of hp0102 were introduced into pBA1-1 by ligation of Eco RI/ Xba I-digested PCR products amplified by CSO-0871/-0872 on gDNA of CSS-0004 and CSO-0309/-0873 on pBA1-1. The resulting plasmid pBA7-4 was used for PCR with oligonucleotides CSO-0870/-0872 and the obtained PCR product was transformed into CSS-0004, CSS-0010, and CSS-0001. Positive erythromycin-resistant clones were checked by PCR on gDNA using CSO-0051 and CSONIH-0033, resulting in strain CSS-1000 (26695 Δ hp0102 ), CSS-1007 (G27 Δ hp0102 ), and CSS-1019 (J99 Δ hp0102 ). Construction of H. pylori LPS mutants in 26695 and X47-2AL Deletion of genes involved in various steps of LPS biosynthesis in H. pylori strains 26695 and X47-2AL were constructed by overlap PCR and subsequent double-crossover homologous recombination. In addition, for strain 26695, new deletion mutants for tlpB , tlpB-hp0102 , and hp0102 carrying the aphA- 3 instead of the rpsL-erm cassette were constructed. Overlap PCR products carried resistance cassettes flanked by ~500 nt of homologous sequence up- and downstream of the gene to be deleted. Resistance cassettes used for cloning were either aphA- 3 (kanamycin) for strain 26695 or aac (3)-IV (apramycin/gentamicin) for X47-2AL. Non-polar resistance cassettes were amplified with HPK1/HPK2 from gDNA of H. pylori strain 26695 C RepG (CSS-0046) [21] , or with CSO-SP008 and CSO-SP009 from pUC1813apra [77] . As an example, deletion of hp1284 in H. pylori strain 26695 will be described in detail. About 500 nt up- and downstream of the hp1284 coding region were amplified using CSO-SP010 × CSO-SP066 and CSO-SP067 × CSO-SP013, respectively. The antisense oligonucleotide of the hp1284 upstream region (CSO-SP066) and the sense oligonucleotide of the hp1284 downstream region (CSO-SP013) contained 21 and 25 nt overlap, respectively, with the sense and antisense oligonucleotide used to amplify the aphA- 3 resistance cassette (HPK1 × HPK2). The final overlap PCR product was amplified with CSO-SP010 and CSO-SP013 using a 1:1:2 ratio of up-/downstream region of hp1284 and aphA- 3 cassette. The program for the overlap PCR was as follows: 1 cycle of [98 °C, 1 min; 61 °C, 1 min; 72 °C, 10 min; 98 °C, 1 min], 40 cycles of [98 °C, 15 s; 57 °C, 30 s; 72 °C, 1 min], followed by 72 °C for 10 min. After size confirmation via agarose gel electrophoresis, the purified PCR product (Macherey-Nagel NucleoSpin PCR cleanup kit) was naturally transformed into the recipient H. pylori 26695 wild-type background (CSS-0004). Kanamycin-resistant clones were verified via colony PCR with CSO-SP014 and HPK2 resulting in the final hp1284 deletion mutant (CSS-5928; ∆ hp1284 ). Deletion mutants for tlpB :: aphA- 3 (CSS-5924; ∆ tlpB (Kan)), tlpB-hp0102 :: aphA- 3 (CSS-5926; ∆ tlpB-hp0102 ), hp0102 :: aphA- 3 (CSS-5942; ∆ hp0102 (Kan)), hp1039 :: aphA- 3 (CSS-5930; ∆ hp1039 ), hp1581 :: aphA- 3 (CSS-5932; ∆ hp1581 ), hp0159 :: aphA- 3 (CSS-5934; ∆ hp0159 ), hp0826 :: aphA- 3 (CSS-5936; ∆ hp0826 ), hp0579-0580 :: aphA- 3 (CSS-5938; ∆ hp0579-580 ), hp1206 :: aphA- 3 (CSS-5940; ∆ hp1206 ) in H. pylori strain 26695, and hp1284 :: aac (3)-IV (CSS-5910; X47-2AL ∆ hp1284 ), hp1039 :: aac (3)-IV (CSS-5912; X47-2AL ∆ hp1039 ), hp1581 :: aac (3)-IV (CSS-5914; X47-2AL ∆ hp1581 ), hp0159 :: aac (3)-IV (CSS-5916; X47-2AL ∆ hp0159 ), hp0826 :: aac (3)-IV (CSS-5918; X47-2AL ∆ hp0826 ), hp0579-0580 :: aac (3)-IV (CSS-5920; X47-2AL ∆ hp0579-580 ), hp1206 :: aac (3)-IV (CSS-5922; X47-2AL ∆ hp1206 ) in H. pylori strain X47-2AL were constructed analogously. Cloning of translational reporter fusions to gfpmut3 For the generation of hp0102 translational reporter fusions, the N-terminal coding region of hp0102 was fused to gfpmut3 and introduced together with the catGC resistance cassette [76] into the rdxA locus of H. pylori strain G27. The first ten amino acids of the hp0102 coding region together with the upstream-encoded gene tlpB , including the tlpB promoter and 5′ UTR (26695, 12G), were amplified from gDNA of H. pylori 26695 (CSS-0004) using oligos CSO-0581/-1803. The purified PCR product was digested with Cla I /Nhe I and ligated with a likewise digested PCR product, which was amplified from pMA5-2 ( cagA 28 th :: gfpmut3 ) using CSO-0146/-0683, resulting in pSP195-6 ( tlpB - hp0102 10 th :: gfpmut3 ). Additional hp0102 10 th :: gfpmut3 reporter fusions were generated by cycle-PCR on pSP195-6 with CSO-1984/-1985 ( tlpB mini - hp0102 ), CSO-2055/-2056 (P tlpB hp0102 ), CSO-2052/-2053 ( tlpB - hp0102 ΔG hp0102 ), CSO-2053/-2061 ( tlpB - hp0102 ATTTA hp0102 ) and CSO-2274/-2275 ( tlpB stop - hp0102 ), respectively. The obtained PCR products were Dpn I - digested, self-ligated, and transformed into E. coli . Positive clones were selected on plates with 100 μg/ml ampicillin and 20 µg/ml chloramphenicol, and confirmed by colony PCR using oligos pZE- Xba I/CSO-0581. The resulting plasmids pSP197-3 ( tlpB mini - hp0102 ), pSP198-4 (P tlpB hp0102 ), pSP200-2 ( tlpB - hp0102 ΔG hp0102 ), pSP201-1 ( tlpB - hp0102 ATTTA hp0102 ), and pSP205-17 ( tlpB stop - hp0102 ) were validated by sequencing with CSO-0206/JVO-0155. Afterwards, these plasmids were used as templates for PCR with CSO-0017/-0018. The PCR products with different hp0102 :: gfpmut3 reporter fusions were transformed into H. pylori G27 wildtype (CSS-0010) and/or Δ repG (CSS-0169). Positive transformants were checked by PCR with CSO-0205/-0207 and the in-frame fusion of hp0102 to gfpmut3 , as well as tlpB , was verified by sequencing with CSO-0206/JVO-0155. The corresponding H. pylori G27 strains are CSS-2104 ( tlpB - hp0102 10 th :: gfpmut3 ), CSS-2107 ( tlpB - hp0102 10 th :: gfpmut3 /Δ repG ), CSS-2116 ( tlpB mini - hp0102 10 th :: gfpmut3 ), CSS-2119 ( tlpB mini - hp0102 10 th :: gfpmut3 /Δ repG ), CSS-2138 (P tlpB hp0102 10 th :: gfpmut3 ), CSS-2141 (P tlpB hp0102 10 th :: gfpmut3 /Δ repG ), CSS-2150 ( tlpB - hp0102 ΔG hp0102 10 th :: gfpmut3 ), CSS-2153 ( tlpB - hp0102 ΔG hp0102 10 th :: gfpmut3 /Δ repG ), CSS-2156 ( tlpB - hp0102 ATTTA hp0102 10 th :: gfpmut3 ), CSS-2159 ( tlpB - hp0102 ATTTA hp0102 10 th :: gfpmut3 /Δ repG ), CSS-3241 ( tlpB stop - hp0102 10 th :: gfpmut3 ) and CSS-3244 ( tlpB stop - hp0102 10 th :: gfpmut3 /Δ repG ). RNA preparation, northern blot, and RT-qPCR If not mentioned otherwise, total RNA from H. pylori grown in liquid culture to mid-exponential growth phase (OD 600 nm of ~0.7–1) was extracted using the hot phenol method as described previously [21] . For northern blot analysis, 5–10 µg total RNA was separated on 6% polyacrylamide (PAA) gels containing 7 M urea and blotted to Hybond-XL membranes (GE-Healthcare). After blotting, total RNA was UV cross-linked to the membrane and hybridized with 5′ end labeled (γ 32 P) DNA oligonucleotides as described previously [21] . For RT-qPCR analysis, RNA samples were digested with DNaseI (Fermentas) to remove genomic DNA. All RT-qPCR experiments were carried out in at least technical and biological triplicates on a CFX96 system (Biorad) using Power SYBR Green RNA-to-C T TM 1-Step kit (Applied Biosystems by Thermo Fisher Scientific) according to the manufacturer’s instructions. Fold-changes were determined by the 2 (−ΔΔCT) -method [79] . The specific primer sets are JVO-5267/-5268 for tlpB mRNA, CSO-0867/-0868 for hp0102 mRNA, and CSO-1173/-1174 for 6S rRNA, which served as internal standard. RT-PCR for verification of the tlpB-hp0102 operon structure For RT-PCR analysis, a DNaseI-digested RNA sample of H. pylori wild-type strain 26695 was reverse transcribed using the High Capacity cDNA Reverse Transcription Kit (Applied Biosystems by Thermo Fisher Scientific, #4368814) according to the manufacturer’s instruction. Briefly, reverse transcriptions were run with 1 µg of RNA ± MultiScribe™ Reverse Transcriptase using the following thermal cycling conditions: [25 °C, 10 min; 37 °C, 120 min; 85 °C, 5 min]. PCR reactions were performed using gene-specific primer sets for tlpB mRNA (JVO-5267/-5268), hp0102 mRNA (CSO-0867/-0868), and for the tlpB-hp0102 operon spanning junction (CSO-SP0061/-0062). PCR amplifications on gDNA of H. pylori wild-type strain 26695 served as a positive control. Subsequently, PCR products were run on a 2% agarose gel. Mouse infection studies H. pylori strain X47-2AL wild-type strain and mutants were used to infect 5-weeks old NMRI-specific pathogen-free female mice (Charles River Laboratories) as published previously in ref. [80] and as described below. The housing conditions of the mice were optimal to reduce their stress. This included half/half light/dark cycle, a constant temperature of 20–23 °C, about 50% humidity, and ad libitum access to water and food. Before infection, the animals underwent an acclimation period of one week. For infections, about 10 8 colony-forming units (CFUs) of H. pylori strains prepared in 100 μl of peptone broth were orogastrically administered to groups of seven mice per strain. In each experiment, four to five mice were inoculated with peptone broth alone as a naive mice negative control. One month after inoculation, mice were sacrificed and stomachs were crushed in peptone broth. CFUs of viable H. pylori bacteria per gram of stomach weight were calculated by serial dilutions and plating on blood-agar plates supplemented with the usual antibiotic-fungicide mixture with, in addition, 200 μg/ml bacitracin and 10 μg/ml nalidixic acid. SDS-PAGE and immunoblotting Cells corresponding to an OD 600 of 1 from H. pylori cells grown to mid-exponential growth phase were collected by centrifugation (16,000 × g at 4 °C for 2 min), resuspended in 100 µl 1× protein loading buffer (62.5 mM Tris-HCl pH 6.8, 100 mM DTT, 10% glycerol, 2% SDS, 0.01% bromophenol blue) and boiled at 95 °C for 8 min. For SDS-PAGE, protein samples corresponding to a total OD 600 of 0.1 were separated by 12% SDS-PAA gels and stained by Coomassie (Fermentas, #R0571). For western blot analysis, protein samples corresponding to an OD 600 of 0.1 or 0.01 were separated by 10–12% SDS-PAGE and transferred to a PVDF membrane by semi-dry blotting. Membranes were blocked for 1 h with 10% milk powder/TBS-T and incubated overnight with primary antibody at 4 °C. After washing with TBS-T, membranes were incubated for 1 h with secondary antibody linked to horseradish peroxidase. Signals were detected using ECL-reagent and Image Quant LAS 4000. To detect the four chemotaxis receptors TlpA, B, C, and D, a polyclonal rabbit TlpA22-antiserum (1:2,000 in 3%BSA/TBS-T) that recognizes a conserved cytosolic domain (kindly provided by Karen Ottemann, University of California, Santa Cruz, CA) and secondary goat anti-rabbit IgG (1:10,000 in 3% BSA/TBS-T; GE-Healthcare, #RPN4301, RRID: AB_2650489) were used. TlpB::3×FLAG was detected by a monoclonal anti-FLAG antibody (1:1,000 in 3% BSA/TBS-T; Sigma-Aldrich, #F1804, RRID: AB_262044) and secondary sheep anti-mouse IgG (1:10,000 in 3% BSA/TBS-T; GE-Healthcare, #RPN4201). GroEL, was visualized by monoclonal anti-GroEL antibody (1:10,000 in 3% BSA/TBS-T; Sigma-Aldrich, #G6532, RRID: AB_259939) and goat anti-rabbit IgG (1:10,000 in 3%BSA/TBS-T). GFP reporter fusion proteins were detected by an anti-GFP antibody (1:1,000 in 3% BSA/TBS-T; Roche, #11814460001) and secondary sheep anti-mouse IgG (1:10,000 in 3% BSA/TBS-T). LPS silver-staining and Lewis x antigen analysis For LPS silver-staining, protein samples were digested with Proteinase K solution (20 mg/ml) for 90–180 min at 60 °C, followed by boiling of the samples for 10 min at 98 °C. Lipopolysaccharide structures from H. pylori were visualized by silver-staining according to ref. [74] . Briefly, LPS samples corresponding to an OD 600 of 0.1 were separated on 15% one dimensional SDS-PAA gel and fixed overnight in 25% isopropanol and 7% acetic acid (1× fixing solution). After incubation in sodium periodate solution (0.7% (w/v) Na 5 IO 6 in 1× fixing solution) for 15 min, gels were washed with water (3 × 30 min). Silver staining solution (0.35% ammonia, 0.02 N NaOH, 0.4% (w/v) silver nitrate) was applied with vigorous agitation for 10 min. Following additional washing steps, gels were developed using a 2.5% (w/v) sodium carbonate solution containing 0.01% (v/v) formaldehyde (37%). Upon completion, 50 mM EDTA was used to stop the development. For western blot analysis of Lewis x/y antigens, LPS samples corresponding to an OD 600 of 0.02 were separated on 15% SDS-PAGE and transferred to a PVDF membrane by semi-dry blotting. Western blot analysis was performed using monoclonal anti-Lewis x antibody (1:500 in 3% BSA/TBS-T, Calbiochem, #434631) and monoclonal anti-Lewis y antibody (1:500 in 3% BSA/TBS-T, Merck, #434636). Chemiluminescence detection was performed with a secondary sheep anti-mouse IgG antibody conjugated to horseradish peroxidase (1:1,000 in 3% BSA/TBS-T, GE Healthcare, #RPN4201). Growth/survival under high salt conditions H. pylori strains were grown in liquid medium (BHI) to exponential growth phase (OD 600 of ~0.7–1.0). Cells were adjusted to an OD 600 of 1.0 in 0.5 ml BHI and serial dilutions of the indicated strains were spotted on GC-agar plates containing sodium chloride at 85 mM (no stress, normal salt content), 200 mM (mild stress), or 260 mM (harsh stress). Plates were incubated for 3–5 days at 37 °C under microaerobic conditions. Antibiotics sensitivity tests The MICs of H. pylori wild-type and mutant strains to polymyxin B were determined in triplicates by Epsilometer (E)-tests (bioMérieux, Inc., #533400) according to the manufacturer’s instructions. Briefly, H. pylori cells corresponding to an OD 600 of 0.1 (exponential growth phase) were spread on GC-agar plates and E-stripes (polymyxin B concentration from 0.064 to 1024 µg/ml) were applied onto the dried surface of the agar plates. MIC values were read from the scale at the intersection of the elliptical zone of inhibition with the graded E-strip after 3 days of incubation under microaerobic conditions at 37 °C. 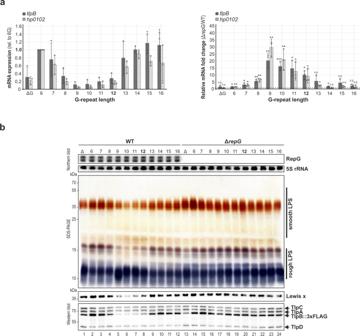Fig. 5: The G-repeat length impacts RepG-mediatedtlpB-hp0102co-regulation and in turn smooth LPS production. a(Left panel) RT-qPCR of relativetlpBandhp0102mRNA levels of differenttlpBleader mutants (ΔG, 6–16G) in theH. pylori26695 wild-type background. The mRNA level of each gene in thetlpB6G-leader mutant was used as reference and set to 1. (Right panel) Relative fold changes oftlpBandhp0102mRNA levels uponrepGdeletion inH. pylori26695tlpBleader mutants when compared to the respective wild-type backgrounds. The fold changes are shown as mean of three biological replicates with corresponding error bars (s.d.). ***—highly significant,p-value < 0.001; **—very significant,p-value < 0.01; *—significant,p-value < 0.05; n.s.—not significant; Student’st-test, two-tailed.bThe LPS patterns and Lewis x antigen levels oftlpBleader mutants inH. pylori26695 wild-type and ∆repGmutant backgrounds were analyzed by silver staining and western blot analysis with anti-Lewis x antigen antibody, respectively. Expression of the chemotaxis receptors was analyzed by an anti-TlpA22 antiserum. Note thattlpBleader mutants express FLAG-tagged TlpB21. A representative silver-stained PAA-gel and western blot are shown (out of three independent experiments). Source data underlying (a,b) are provided as a Source data file. 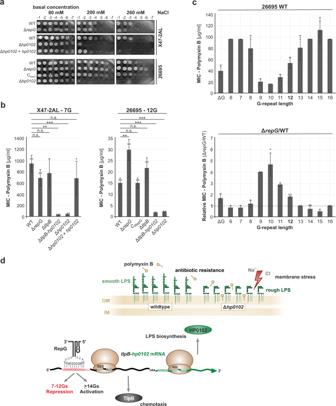Fig. 6: RepG affects sensitivity to salt stress and polymyxin B via regulation ofhp0102. aH. pyloriX47-2AL and 26695 WT and indicated mutant strains were grown in liquid culture to exponential growth phase (OD600of 1). Indicated ten-fold dilutions of the bacterial suspensions were spotted on GC-agar plates containing 80 mM (basal concentration), 200 mM (mild stress), or 260 mM (harsh stress) sodium chloride. Plates were incubated for 3–5 days at 37 °C under microaerobic conditions. The results shown are representative of at least two independent experiments.bPolymyxin B sensitivity testing forH. pyloriX47 and 26695 WT and indicated mutant strains using E-tests. Error bars indicate s.d. forn= 3 independent biological experiments. ****— highly significant,p-value < 0.0001; **—very significant,p-value < 0.01; n.s.—not significant; Student’st-test, two-tailed.c(Upper panel) Polymyxin B MICs ofH. pylori26695tlpBmRNA leader variants in the wild-type background. (Lower panel) Relative fold changes in polymyxin B sensitivity (MICs) uponrepGdeletion in differenttlpBleader variants when compared to the respective wild-type backgrounds (n= 2 for WT/∆repG_∆G, ∆repG_6G, WT/∆repG_7-9G, WT/∆repG_11G, WT/∆repG_13G, WT/∆repG_15-16G;n= 3 for WT_6G, WT/∆repG_10G, WT/∆repG_12G, WT/∆repG_14G).dModel of RepG-mediated regulation of TlpB and HP0102. The genes encoding the chemotaxis receptor TlpB (dark gray) and the fucosyltransferase HP0102 (green) are transcribed as a bicistronic mRNA and play a role in chemotaxis25and smooth LPS biosynthesis (light green) as well as protection against membrane stress (indicated by red arrow), respectively. Deletion ofhp0102leads to loss of O-antigens and a rough LPS phenotype (dark green). Antisense base-pairing of the C/U-rich terminator loop of RepG sRNA to the homopolymeric G-repeat in the 5′ UTR of thetlpB-hp0102mRNA results in post-transcriptional co-regulation oftlpBandhp0102at the transcript and protein level. Depending on the G-repeat length, RepG mediates both repression (7–12Gs) and activation (≥14Gs) oftlpBandhp0102. OM/IM—outer/inner membrane, RBS—ribosome binding site, AUG/UUG—start codons, UAA—stop codon. Source data underlying (b,c) are provided as a Source data file. E-test MICs that were between the standardized two-fold dilution steps were rounded to the next higher concentration. Biocomputational search for repG , tlpB , and hp0102 homologs Using BLAST (Basic Local Alignment Search Tool, NCBI) and SyntTax webserver ( https://archaea.i2bc.paris-saclay.fr/SyntTax/ ), biocomputational searches for repG , tlpB , and hp0102 homologs were performed in diverse Helicobacter species (spp.) and other related Epsilonproteobacteria, including Campylobacter spp., Wolinella spp., Sulfuricurvum spp., Arcobacter spp., Sulfurospirillum spp., and Nautilia profundicola (~120 genomes). Genes were considered to be homologous when they share more than 30% percent sequence similarity with repG , tlpB , and hp0102 of H. pylori strain 26695. No homologs for repG, tlpB , and hp0102 could be identified outside of the Helicobacter spp. and thus, are not further mentioned in the main text. Ethics Statement Experiments in mice were carried out in strict accordance with the recommendations in the Specific Guide for the Care and the Use of Laboratory Animals of the Institut Pasteur, according to the European Directive (2010/63/UE) and the corresponding French law on animal experimentation (Arrêtés de 1988). The protocol has been approved by the Committee of Central Animal Facility Board of the Institut Pasteur. To follow the new European directives, the project was approved by the CETEA, Comité d’éthique en Expérimentation Animale of the Institut Pasteur (#2013-0051) and by the Ministère de l’Enseignement Supérieur et de la recherche (#751501). Reporting summary Further information on research design is available in the Nature Research Reporting Summary linked to this article.